Parasympathetic stimulation improves epithelial organ regeneration Parasympathetic nerves are a vital component of the progenitor cell niche during development, maintaining a pool of progenitors for organogenesis. Injured adult organs do not regenerate after parasympathectomy, and there are few treatments to improve organ regeneration, particularly after damage by therapeutic irradiation. Here we show that restoring parasympathetic function with the neurotrophic factor neurturin increases epithelial organ regeneration after damage. We use mouse salivary gland explant culture containing fluorescently labelled progenitors, and injure the tissue with irradiation. The progenitors survive, parasympathetic function is diminished and epithelial apoptosis reduces the expression of neurturin, which increases neuronal apoptosis. Treatment with neurturin reduces neuronal apoptosis, restores parasympathetic function and increases epithelial regeneration. Furthermore, adult human salivary glands damaged by irradiation also have reduced parasympathetic innervation. We propose that neurturin will protect the parasympathetic nerves from damage and improve organ regeneration. This concept may be applicable for other organs where parasympathetic innervation influences their function. Tissue regeneration occurs in many lower organisms after damage [1] , [2] and classic experiments demonstrate the importance of peripheral nerves for amphibian muscle and limb regeneration [3] . The peripheral nerves are composed of parasympathetic and sympathetic branches of the autonomic nervous system. Nerves from the parasympathetic branch are critical for the function of the gastrointestinal tract, urogenital organs, trachea, cornea, prostate, exocrine pancreas, and lacrimal and salivary glands. Parasympathetic innervation also influences organ regeneration: tissue regrowth is impaired after parasympathectomy in the salivary gland [4] . Injured adult organs also do not regenerate after damage by therapeutic irradiation (IR), despite the presence of stem and progenitor cells [5] , [6] , [7] , [8] . Thus, we hypothesized that after organ damage by IR the surviving progenitors do not regenerate the organ because of altered parasympathetic innervation and function. To test this hypothesis, we used the fetal mouse submandibular salivary gland (SMG) for a number of reasons. The SMG epithelium develops by branching morphogenesis and this occurs in parallel with the migration of axon bundles from the parasympathetic submandibular ganglion (PSG) towards the end bud epithelium [9] , [10] . Parasympathetic innervation during development maintains undifferentiated keratin 5-positive (K5+) epithelial progenitors that are required for salivary gland organogenesis [9] . Importantly, sympathetic innervation occurs around birth, allowing us to study the parasympathetic innervation in isolation. In addition, there is a clinical need to improve salivary gland function after the permanent IR damage that occurs during head and neck cancer therapy [8] . Neurturin (NRTN) is an important neurotrophic factor involved in parasympathetic nervous system function and survival; it binds its receptor GFRα2 and signals via RET, a tyrosine kinase coreceptor, and Src-kinase [11] , [12] . Importantly, Nrtn −/− , Gfra2 −/− and Ret −/− mice have smaller parasympathetic ganglia and multiple defects in epithelial function owing to reduced innervation of the gastrointestinal and reproductive tracts, lacrimal and salivary glands [13] , [14] , [15] , [16] . To investigate the role of parasympathetic innervation during organ regeneration, we used fetal SMG explant culture from K5-venus transgenic mice, which have fluorescent K5+ cells [9] , and damaged the tissue with gamma IR. This results in epithelial apoptosis and reduced innervation but the K5+ progenitor cells remain. Here, we show that NRTN, which is produced by the SMG epithelium during development, restores parasympathetic innervation and promotes epithelial regeneration after IR. In addition, we show that adult human salivary glands damaged by IR also have a reduction in parasympathetic innervation. We speculate that NRTN may be useful to protect or restore parasympathetic function to reduce IR damage and improve organ regeneration. IR reduces parasympathetic innervation by apoptosis Exposing embryonic day 13 (E13) SMGs to IR (5 Gy) reduced epithelial morphogenesis; after 5 days the end bud number was reduced by ~80% and ductal structures remained ( Fig. 1a ). There were ~30% less PSG axons compared with control, which still extended along the epithelium, and K5+ progenitors survived ( Fig. 1a ). The loss of epithelial end buds in E13 SMGs after 5 Gy IR was due to substantial apoptosis, which occurred in ~30% of end bud cells and ~1% of PSG neurons within 24 h ( Supplementary Fig. S1 ). An increase in IR dose (7 Gy) reduced epithelial morphogenesis by ~90% and there was a striking reduction of innervation with ~80% fewer axons, although multiple small ganglia survived ( Fig. 1a , arrowheads). The surviving epithelium contained mostly K5+ progenitors ( Fig. 1a–b ) and K19+ cells: K19 is a marker of ductal differentiation [9] ( Supplementary Fig. S2 ). Supporting these findings, gene expression analysis 3 days after 7 Gy IR ( Fig. 1c ) showed increased expression of Krt5 , Krt19 , Egfr and its ligand Hbegf . Hbegf binds Egfr and stimulates K5 cells to differentiate along the duct lineage and express K19 (ref. 9 ). IR also reduced the expression of neuronal tubulin ( Tubb3 ), an axonal marker in the parasympathetic nerves, that have been previously shown to effect epithelial progenitor cell maintenance [9] . Furthermore, there was reduced expression of the water channel aquaporin 5 ( Aqp5) , a marker of end bud differentiation and Fgf1 , a component of the FGFR signalling pathway that is essential for epithelial survival and proliferation [17] ( Fig. 1c ). These data demonstrate that E13 SMGs are sensitive to IR, which reduced end bud morphogenesis via apoptosis, decreased parasympathetic innervation and increased ductal K19+ cell differentiation. To further define the temporal sequence of apoptotic events, we measured cleaved caspase-3 (Casp3) in the PSG and the epithelium of irradiated E14 SMGs at 1, 3 and 5 days (D) after 5 Gy IR ( Supplementary Fig. S2 ). We used E14 SMGs as 5 Gy IR results in less epithelial apoptosis within 24 h. These data show decreasing epithelial apoptosis with time: ~13% of E14 epithelial cells undergo apoptosis within 1 day, ~6% at D3 and <0.3% by D5. Both K19− and K19+ cells undergo apoptosis indicating that progenitor cells of the ductal lineage are equally sensitive to IR-induced cell death as other epithelial lineages. In contrast to the epithelial compartment, apoptosis of the PSG increased with time from 1% of cells at D1 to ~5% of cells at D3. The extensive rapid epithelial apoptosis at D1 post IR combined with reduced PSG innervation and increased neuronal cell death by D3 led us to predict that the epithelium produced neurotrophic factors that helped maintain functional innervation. 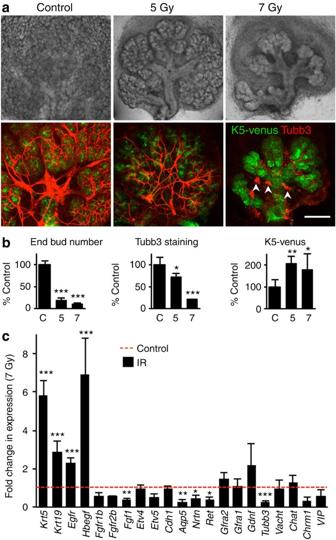Figure 1: IR decreases epithelial morphogenesis and parasympathetic innervation. (a) Submandibular glands (SMG) from E13 K5-venus transgenic mice irradiated (IR dose of 5 and 7 Gy) and cultured for 5 days. Whole-mount images of K5-venus and nerves (Tubb3) are shown. Arrows point to ducts and arrowheads point to small ganglia. Scale bar, 200 μM. (b) Quantitation of epithelial morphogenesis (end bud number), innervation (Tubb3 fluorescence) and K5+ progenitors (K5-venus fluorescence) were quantitated and normalized to the control (C=100%). Three to five SMGs were used per group and experiments repeated three times, see SOM for details. A one-way analysis of variance withpost hocDunnett’s test; ***P<0.001, **P<0.01, *P<0.05. (c) qPCR analysis of gene expression in E13 SMGs 3 days after 7 Gy IR compared with control. Means±s.d. from three experiments. A false discovery rate (Q) for multiple unpairedt-tests was set to 5%; ***P<0.001, **P<0.01, *P<0.025. Figure 1: IR decreases epithelial morphogenesis and parasympathetic innervation. ( a ) Submandibular glands (SMG) from E13 K5-venus transgenic mice irradiated (IR dose of 5 and 7 Gy) and cultured for 5 days. Whole-mount images of K5-venus and nerves (Tubb3) are shown. Arrows point to ducts and arrowheads point to small ganglia. Scale bar, 200 μM. ( b ) Quantitation of epithelial morphogenesis (end bud number), innervation (Tubb3 fluorescence) and K5+ progenitors (K5-venus fluorescence) were quantitated and normalized to the control (C=100%). Three to five SMGs were used per group and experiments repeated three times, see SOM for details. A one-way analysis of variance with post hoc Dunnett’s test; *** P <0.001, ** P <0.01, * P <0.05. ( c ) qPCR analysis of gene expression in E13 SMGs 3 days after 7 Gy IR compared with control. Means±s.d. from three experiments. A false discovery rate ( Q ) for multiple unpaired t -tests was set to 5%; *** P <0.001, ** P <0.01, * P <0.025. Full size image NRTN increases parasympathetic neuronal function In order to identify epithelial-derived neurotrophic factors, we analysed E13 epithelium separated from mesenchyme by microarray. We identified 473 genes more highly expressed (5-fold, P <0.001) in the epithelium than the mesenchyme. Using the Gene Ontology term: Nervous system development (GO:0007399), we narrowed this to 36 genes, 2 of which were secreted neurotrophic factors, NRTN and neurotrophin 5 ( Supplementary Table S1 ). Of these two, only NRTN is involved in parasympathetic nervous system function; it binds GFRα2 and signals via RET coreceptor and Src-kinase [12] , [13] . We confirmed that NRTN was expressed in SMG epithelium, GFRα2 in the nerves and Ret was localized in the PSG surrounding the duct ( Supplementary Fig. S3A –C). As predicted, IR reduced the expression of Nrtn and also reduced Ret by ~2-fold but did not change GFRa2 expression ( Fig. 1c ). These data suggest that IR-induced epithelial apoptosis decreases NRTN expression, which reduces parasympathetic innervation. We then hypothesized that NRTN-dependent PSG axon outgrowth and function would influence epithelial morphogenesis. To test this hypothesis, we used both isolated PSG and SMG explant cultures. In gain-of-function experiments, we cultured isolated PSG in a three-dimensional laminin matrix with a bead soaked in recombinant NRTN. Neurites extended towards the NRTN bead ( Fig. 2a ) and increased the number of varicosities (unconventional synapses) that release neurotransmitters ( Fig. 2b ). NRTN signals via the Gfrα2/Ret/Src–kinase complex [18] , and NRTN-dependent neurite outgrowth was abrogated by a Src-kinase inhibitor ( Supplementary Fig. S4A ). We also tested the effects of other neurotrophic factors on PSG neurite outgrowth. Only GDNF, which also binds GFRα2, stimulated neurite outgrowth similar to NRTN while the other factors were similar to control ( Supplementary Fig. S4B ). NRTN reduced neuronal apoptosis ( Supplementary Fig. S4C ) and increased the expression of genes involved in parasympathetic function within 24 h, including Gfra2 (1.5-fold), Ret (~10-fold), Tubb3 (~5-fold), Vacht (1.6-fold), synapsin II ( Syn2 , 4-fold), Ncam (1.6-fold) and L1cam (3-fold), while chromogranin ( Chg ) expression did not change ( Fig. 2c ). In loss-of-function experiments, a function-blocking NRTN antibody [19] reduced morphogenesis by ~40%, neuronal outgrowth by ~30% and the number of varicosities by ~90% compared with control ( Fig. 2d ). Together, these data supported our hypothesis that NRTN-dependent parasympathetic outgrowth and function modulate morphogenesis. 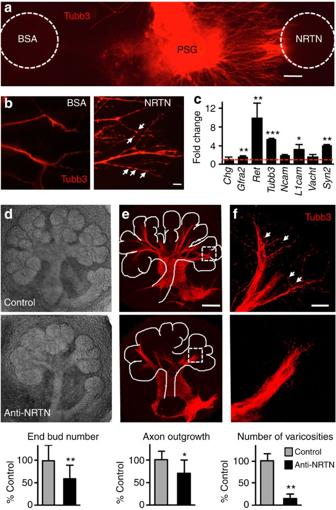Figure 2: NRTN increases parasympathetic neurite outgrowth and function. (a) Whole-mount image (Tubb3 staining) of a PSG cultured with a BSA and a NRTN-coated bead. Scale bar, 100 μm. (b) Higher magnification of neurites to show varicosities (arrows). Scale bar, 20 μm. (c) qPCR analysis of gene expression in PSGs treated with NRTN. Data were normalized toRps29and BSA-treated PSGs. (d) Images of SMGs cultured with a function-blocking NRTN antibody or an IgG control. Epithelial morphogenesis (end bud number) was quantitated and normalized to IgG control. (e) Whole-mount staining of the nerves. Axon outgrowth was measured using Tubb3 fluorescence and normalized to epithelial area, see SOM for details. Scale bar, 100 μm. (f) Higher magnification of nerves highlights the varicosities. The number of varicosities was counted. Scale bar, 20 μm. All graphs are all normalized to the IgG control. Means±s.d. from three experiments. Student’st-test; ***P<0.001, **P<0.01, *P<0.05. Figure 2: NRTN increases parasympathetic neurite outgrowth and function. ( a ) Whole-mount image (Tubb3 staining) of a PSG cultured with a BSA and a NRTN-coated bead. Scale bar, 100 μm. ( b ) Higher magnification of neurites to show varicosities (arrows). Scale bar, 20 μm. ( c ) qPCR analysis of gene expression in PSGs treated with NRTN. Data were normalized to Rps29 and BSA-treated PSGs. ( d ) Images of SMGs cultured with a function-blocking NRTN antibody or an IgG control. Epithelial morphogenesis (end bud number) was quantitated and normalized to IgG control. ( e ) Whole-mount staining of the nerves. Axon outgrowth was measured using Tubb3 fluorescence and normalized to epithelial area, see SOM for details. Scale bar, 100 μm. ( f ) Higher magnification of nerves highlights the varicosities. The number of varicosities was counted. Scale bar, 20 μm. All graphs are all normalized to the IgG control. Means±s.d. from three experiments. Student’s t -test; *** P <0.001, ** P <0.01, * P <0.05. Full size image NRTN improves regeneration after IR We then predicted that NRTN would reduce neuronal apoptosis, restore parasympathetic function and improve epithelial regeneration after IR. To test this prediction, we irradiated E14 SMGs with either 5 Gy or 7 Gy, added recombinant NRTN (1 ng ml −1 ), and measured epithelial regeneration and neuronal apoptosis and function 3 days later. As predicted, NRTN increased the number of end buds after IR >2-fold ( Fig. 3a–e ). The nerves extended along the epithelium ( Fig. 3b ); there was an increase in Ecadherin (Ecad)+K5–K19− end buds ( Fig. 3c and Supplementary Fig. S5A , red cells); a reduction in neuronal apoptosis ( Fig. 3d ); and an increase in end bud number with both doses of IR ( Fig. 3e ). Although the increase in end bud number was similar with both doses of IR, the epithelium treated with 7 Gy was more severely damaged and Ecad immunostaining was reduced, although still present, throughout the epithelium (see higher magnification in Supplementary Fig. S5A ). NRTN did not increase epithelial morphogenesis in non-IR SMGs ( Supplementary Fig. S5B ). NRTN restored the expression of genes involved in parasympathetic axon outgrowth and function to control levels, such as Tubb3 , Vacht , Chat and Ret , while Gfra2 expression, the receptor for NRTN, did not change. NRTN also increased expression of Cdh1, Fgfr1b , Etv4 and Etv5 and rescued Fgf1 expression ( Fig. 3f ) indicating epithelial end bud proliferation had increased. In addition, expression of p21 , a marker of cell cycle arrest, increased with IR and returned to control levels with NRTN suggesting that cells had reentered the cell cycle. Expression of Krt5 , Krt19 , Egfr and Hbegf , genes associated with ductal differentiation, were higher than control after IR, and NRTN did not alter their expression. To examine whether increased bud formation was in part owing to ACh release, IR-SMG were treated with the ACh analogue carbachol (CCh). Treatment of IR-SMG with CCh (10 nM) increased morphogenesis but higher doses (100 nM) did not ( Supplementary Fig. S5C ), suggesting that dose-dependent cholinergic signalling is involved in regeneration after IR. In contrast, treatment with nerve growth factor (NGF) did not increase morphogenesis ( Supplementary Fig. S5C ). NRTN may stimulate the release of other factors from the nerves, apart from ACh, and these remain to be determined. In summary, exogenous NRTN reduces neuronal apoptosis and restores parasympathetic function, which promotes regeneration. 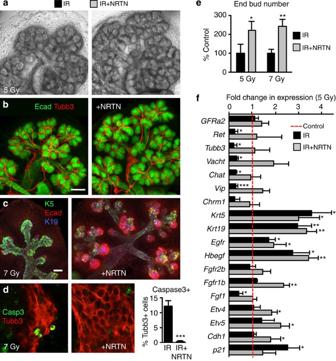Figure 3: NRTN treatment reduces neuronal apoptosis and restores parasympathetic function. (a) SMGs from E14 mice were irradiated with 5 Gy, treated with NRTN (1 ng ml−1) and cultured for 3 days. (b) Whole-mount images of the epithelium (Ecad) and nerves (Tubb3) are shown. Scale bar, 100 μm. (c) E14 SMGs were irradiated with 7 Gy, cultured 3 days and stained for epithelium (Ecad), K5+ cells and K19+ cells (also seeSupplementary Fig. S5A). Scale bar, 50 μm. (d) Neuronal apoptosis was measured in E14 SMGs treated with 7 Gy IR for 3 days by Casp3 staining and the percentage of Casp3+Tubb3+ cells measured. Means±s.d. from three experiments. Student’st-test; ***P<0.001. (e) Epithelial morphogenesis (end bud number) was quantitated and normalized to IR SMG. Means±s.d. from three experiments. Student’st-test; **P<0.01, *P<0.05. (f) qPCR analysis after 3 days culture of control and 5 Gy IR +/− NRTN treatment. Data were normalized toRps29and non-IR control. Mean±s.d. of three independent experiments. A one-way analysis of variance withpost hocDunnett’s test; *P<0.05, **P<0.01, ***P<0.001. Figure 3: NRTN treatment reduces neuronal apoptosis and restores parasympathetic function. ( a ) SMGs from E14 mice were irradiated with 5 Gy, treated with NRTN (1 ng ml −1 ) and cultured for 3 days. ( b ) Whole-mount images of the epithelium (Ecad) and nerves (Tubb3) are shown. Scale bar, 100 μm. ( c ) E14 SMGs were irradiated with 7 Gy, cultured 3 days and stained for epithelium (Ecad), K5+ cells and K19+ cells (also see Supplementary Fig. S5A ). Scale bar, 50 μm. ( d ) Neuronal apoptosis was measured in E14 SMGs treated with 7 Gy IR for 3 days by Casp3 staining and the percentage of Casp3+Tubb3+ cells measured. Means±s.d. from three experiments. Student’s t -test; *** P <0.001. ( e ) Epithelial morphogenesis (end bud number) was quantitated and normalized to IR SMG. Means±s.d. from three experiments. Student’s t -test; ** P <0.01, * P <0.05. ( f ) qPCR analysis after 3 days culture of control and 5 Gy IR +/− NRTN treatment. Data were normalized to Rps29 and non-IR control. Mean±s.d. of three independent experiments. A one-way analysis of variance with post hoc Dunnett’s test; * P <0.05, ** P <0.01, *** P <0.001. Full size image IR reduces parasympathetic innervation in human SMGs To determine whether a reduction in parasympathetic function also occurs in IR adult human SMGs, we analysed SMG biopsies from patients irradiated during head and neck cancer treatment ( n =3) and compared them with non-IR controls ( n =5). Thick frozen sections (100 μm) of the biopsy specimens were used for immunostaining, allowing us to visualize the axons within the tissue by projecting multiple optical sections. RNA was isolated from 150 μm frozen sections of the same biopsies as described in the Methods. K5+ cells are present in the epithelium of both non-IR and IR biopsies. Ducts (d, in Fig. 4a ) are abundant compared with acinar structures (a) in IR SMGs as previously reported [20] and these results are similar to our findings in the mouse fetal SMG ( Fig. 1a , arrows). As predicted by the mouse studies, both NRTN (immunolocalized in remaining epithelial cells; Fig. 4b ) and parasympathetic nerves, as measured by GFRα2 staining ( Fig. 4c ), were reduced by ~60% in IR human SMGs. However, gene expression of NRTN , GFRA2 and VIP did not change after IR, although there was reduced expression of CHRM1 , CHRM3 and AQP5 , and increased expression of KRT5 , KRT19, EGFR and HBEGF , consistent with the effects of IR on mouse fetal SMGs ( Fig. 4e ). GFRα2 is also expressed on Schwann cells, which do not express Tubb3, and NRTN could potentially affect Schwann cell function after IR, although this remains to be determined. Surprisingly, there was increased Tubb3 immunostaining ( Fig. 4c ) and TUBB3 gene expression ( Fig. 4e ) after IR, which was likely the result of increased sympathetic innervation. Accordingly, there was increased tyrosine hydroxylase staining ( Fig. 4c ) and increased expression of markers of sympathetic innervation, including the alpha 2B adrenergic receptor , NGF and its receptor, and the neurotrophic tyrosine kinase receptor-1 ( Fig. 4e ). Although the irradiated human salivary glands were compared to unirradiated, unrelated control salivary glands, these data suggest that IR of SMGs disrupts the balance of parasympathetic and sympathetic innervation to the salivary glands. 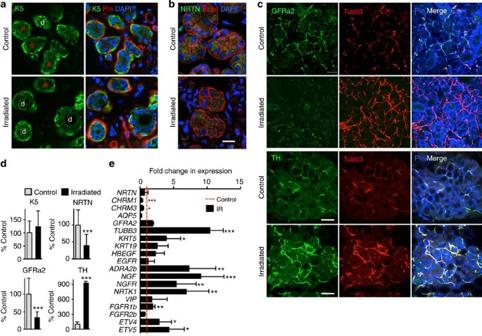Figure 4: IR of adult human SMGs reduces parasympathetic innervation. (a) Control non-IR and IR SMGs were immunostained for K5; the basement membrane was stained with perlecan (Pln) and the nuclei with 4,6-diamidino-2-phenylindole. Acinar units (a) and ducts (d) are labelled in the K5 images. (b) NRTN immunostaining is in the epithelium (Ecad). Nuclei are stained with 4,6-diamidino-2-phenylindole. Images are single confocal sections (2 μm), scale bar, 20 μm. (c) GFRa2 immunostaining labels the parasympathetic nerves, tyrosine hydroxylase (TH) labels sympathetic nerves, Perlecan (Pln) labels the basement membrane and Tubb3 is a pan-neuronal marker. Images are single confocal projections (20 μm), scale bar, 50 μm. (d) K5, NRTN, GFRa2 and TH fluorescence was quantitated; K5, GFRa2 and TH were normalized to perlecan, which stains IR and control tissues at a similar level, but NRTN was normalized to Ecad to show that the remaining epithelium produces less NRTN, and all were expressed as a percentage of non-IR control. (e) qPCR analysis of gene expression normalized toGAPDHand non-IR control. Mean±s.d. of IR (n=3) and non-IR human SMGs (n=5). A false discovery rate (Q) for multiple unpairedt-tests was set to 5%; ***P<0.001, **P<0.01, *P<0.025. Figure 4: IR of adult human SMGs reduces parasympathetic innervation. ( a ) Control non-IR and IR SMGs were immunostained for K5; the basement membrane was stained with perlecan (Pln) and the nuclei with 4,6-diamidino-2-phenylindole. Acinar units (a) and ducts (d) are labelled in the K5 images. ( b ) NRTN immunostaining is in the epithelium (Ecad). Nuclei are stained with 4,6-diamidino-2-phenylindole. Images are single confocal sections (2 μm), scale bar, 20 μm. ( c ) GFRa2 immunostaining labels the parasympathetic nerves, tyrosine hydroxylase (TH) labels sympathetic nerves, Perlecan (Pln) labels the basement membrane and Tubb3 is a pan-neuronal marker. Images are single confocal projections (20 μm), scale bar, 50 μm. ( d ) K5, NRTN, GFRa2 and TH fluorescence was quantitated; K5, GFRa2 and TH were normalized to perlecan, which stains IR and control tissues at a similar level, but NRTN was normalized to Ecad to show that the remaining epithelium produces less NRTN, and all were expressed as a percentage of non-IR control. ( e ) qPCR analysis of gene expression normalized to GAPDH and non-IR control. Mean±s.d. of IR ( n =3) and non-IR human SMGs ( n =5). A false discovery rate ( Q ) for multiple unpaired t -tests was set to 5%; *** P <0.001, ** P <0.01, * P <0.025. Full size image The present study has uncovered a novel mechanism for promoting regeneration of tissue damaged by IR. We previously found that the parasympathetic nerves were necessary for maintaining K5+ epithelial progenitor cells during development. Here, we show that the parasympathetic neuronal function promotes tissue regeneration after IR in the salivary gland and that the epithelium produces a neurotrophic factor that maintains the nerves. There is a substantial loss of the secretory acinar epithelium in humans after IR of their salivary glands during cancer treatment. Our data suggest that this loss of acinar cells may also result in reduced parasympathetic innervation, thus further compromising salivary function and regeneration. Indeed, the anatomy of gland innervation may in part explain the effects of IR on autonomic nerves. As the cell bodies of the PSG are located within the gland, they may be more affected by IR, whereas the sympathetic nerves cell bodies are located in the superior cervical ganglion, and may be distant from the site of IR. Whether IR causes PSG apoptosis in humans, as occurs in IR fetal mouse SMGs, remains to be determined. In addition, sympathetic nerves regulate salivary secretion but are not present during early SMG development and may have inhibitory effects on epithelial regeneration, as sympathetic signalling blocks muscarinic-induced EGFR activation [21] . In the SMG, increased sympathetic activity would likely result in reduced progenitor cell self-renewal [9] . For example, blocking sympathetic function increases hepatic progenitors and liver regeneration [22] . It may be that reduced parasympathetic function combined with increased sympathetic innervation after IR negatively influences organ regeneration. In conclusion, we propose that epithelial organ regeneration can occur after injury if parasympathetic innervation is maintained. Without functional innervation and the factors that maintain neuronal–epithelial communication, regeneration does not occur. We speculate that NRTN treatment may protect parasympathetic neurons and/or increase their function, which would prevent or reduce IR damage and improve regeneration with or without additional stem cell therapy. This may be important in a number of organs with parasympathetic innervation that also express NRTN, including the gastrointestinal tract, trachea, cornea, exocrine pancreas, lacrimal glands and hair follicles [23] . NRTN is an attractive candidate for gene therapy to improve epithelial organ regeneration, as a NRTN-expressing adeno-associated virus is currently in gene therapy trials to improve motor function of patients with Parkinsons disease [24] . Keratin 5-venus mice The K5-venus-expressing transgenic mouse has been previously described [9] . The 5.4 kb bovine K5 promoter, which includes 5′ regulatory and promoter regions from −5,300 bp to +138 bp, directs Venus (YFP variant) expression to epithelia analogous to endogenous K5 (ref. 25 ). The expression of the K5-venus was previously compared with endogenous K5 expression by staining SMGs from K5-venus mice, with both anti-K5 and anti-EGFP antibodies, which recognize Venus [9] . Ex vivo SMG culture and IR Fetal SMG explants from either K5-venus or ICR embryos were cultured as previously described [26] . E13 or E14 SMGs or PSGs (see below) were placed in culture dishes and irradiated in a Gammacell 1000 irradiator with a single dose of IR. Following IR, SMGs were incubated with fresh medium containing bovine serum albumin (BSA), NRTN (1, 10 and 100 ng ml −1 ; the optimal dose was determined to be 1 ng ml −1 ), CCh (0.1, 1, 10 and 100 nM, C4382, Sigma) or NGF (1, 10, and 100 ng ml −1 ) and the SMGs cultured for a further 24–72 h. Explants were either lysed for RNA or fixed for immunostaining. E12 SMGs from ICR mice were cultured for 48 h and a neutralizing antibody to mouse neurturin (AB477; R&D Systems) or goat IgG control antibody (sc2028-L; Santa Cruz Biotechnology) was added to the media at 50 μg ml −1 . The end bud number was counted at the beginning of the experiment (Time 0) and at the end of the assay and expressed as a ratio (End point/T0), and normalized to the control treatment (% control). All experiments showing end bud number were obtained using 3–5 SMGs per group and each experiment repeated at least three times. PSG explant culture PSGs were dissected from E13 SMG using dispase treatment and mechanical dissection, and placed in 15 μl of laminin-111 (Trevigen) on a 0.1 μm Nucleopore filter floating above serum-free media. Medium was supplemented with NRTN (10 and 100 ng ml −1 ; R&D Systems) or 0.1% BSA. PSG were cultured for 24 h for neurite outgrowth assays, and 90 h for survival assays. In some assays, cultures were incubated with chemical inhibitors to PI3K (LY294002, 25 mM), MAPK (UO126, 20 mM) and Src-kinase (PP2, 5 mM; Calbiochem). PSGs were lysed for quantitative PCR (qPCR) analysis or fixed for immunofluorescence analysis. PSGs were also cultured with BSA, NRTN, glial cell line-derived neurotrophic factor GDNF, brain-derived neurotrophic factor, artemin, persephin, ciliary neurotrophic factor, (neurotrophin-3) NT-3 or NGF β (all at 10 and 100 ng ml −1 ). For bead assays, a protocol was adapted from Thesleff and Sahlberg [27] . Acrylic heparin beads (Sigma) were incubated with 30 μl NRTN (10 μg ml −1 in 0.1% BSA; R&D Systems) or 0.1% BSA at 37 °C for 45 min, centrifuged briefly and rinsed with PBS. Beads were placed in laminin matrix using a pipette. Gene expression analysis Real-time PCR was performed as previously described [28] . Primers were designed using Beacon Designer software. Melt curves and primer efficiency were determined as previously described. Gene expression was normalized to Rps29 or GAPDH and to the corresponding experimental control, and reactions were run in triplicate and repeated three times. Immunofluorescence and in situ analysis Whole-mount SMG immunofluorescence analysis has been described [9] . SMGs and PSGs were fixed with 4% paraformaldehyde for 20 min at room temperature and/or ice cold acetone/methanol for 5 min. Tissue was blocked for 1–3 h with 10% Donkey Serum (Jackson Laboratories, ME), 1% BSA and MOM IgG-blocking reagent (Vector Laboratories, CA) in 0.01% PBS-Tween-20. The SMGs were incubated with primary antibodies overnight at 4 °C: goat anti-GFRa2 (1:100; R&D systems), goat anti-neurturin (AB477, 1:100; R&D systems), mouse anti-Tubb3 (clone TUJ1 at 1:200; R&D Systems), cytokeratin 5 (AF 138 at 1:1200; Covance Research); rabbit anti-Caspase-3 (1:200; Cell Signaling) and mouse anti-Ecadherin (1:200; BD Transduction). Nuclei were stained with To-pro3, 4,6-diamidino-2-phenylindole or Hoechst. Antibodies were detected using Cy2-, Cy3- or Cy5-conjugated secondary Fab fragment antibodies (Jackson Laboratories). Fluorescence was analysed using a Zeiss 710 LSM microscope (Zeiss). Quantitation of Tubb3 and K5-venus fluorescence in SMG culture was calculated from a single projection of confocal images through the intact SMG ( n =3). The Tubb3 expression was normalized to the epithelial area, and expressed as a percentage of control treatment. Apoptosis was analysed by Casp3 immunostaining of E14 SMGs treated with 5 GY IR at D1, D3 and D5 ( n =3 for each group). SMGs were immunostained for Casp3, Keratin 19 (K19) and either Ecad or beta3-Tubb3, and the number of apoptotic cells within the K19+, K19− epithelial cells, and the PSG cell bodies were counted. We used 12 × 5 μm 2 sections of three separate end buds in each gland, three secondary ducts, the primary duct and the PSG. We counted the number of Casp3+ cells in every fourth section of each stack ( n =3 section per area), and the number of other cells (either K19+, Ecad+ or Tubb3+) in the section. The PSG apoptosis was in the Tubb3+ cell bodies of the ganglion. Whole-mount in situ hybridization was performed on isolated E13 SMGs as previously described [29] . Axon outgrowth and varicosity measurements The extent of axon outgrowth and varicosity formation in cultured SMGs was quantified using immunofluorescent images and ImageJ software (NIH, http://rsbweb.nih.gov/ij/ ). Axon outgrowth was measured after Tubb3 immunostaining using a single projection of confocal images through the intact SMG ( n =5), and the length of the axon bundles from the ganglia towards the end bud was normalized to the area of the epithelium. The experiment was repeated and the results combined. Varicosities (punctate structures <2 μm in diameter) were counted within 5 × 50 μm 2 fields placed randomly at the end of axon bundles. Microarray analysis Agilent whole-mouse genome microarray analysis (Agilent) was performed as described in the manufacturers instructions. E13 SMGs were separated into epithelia and mesenchymal cells, and four independent pools of RNA were made from each cell type. Arrays were analysed with Genespring Software, identifying genes with a >5-fold difference in expression and a P -value <0.001. Genes were filtered by Gene Ontology Analysis Software and we focused on genes expressed in the epithelium that were present in the term GO:0007399; Nervous system development. The array data are available in the SGMAP Database (Salivary Gland Molecular Anatomy Project, http://sgmap.nidcr.nih.gov/sgmap ). Analysis of human biopsy tissue Human SMG tissue samples from patients with an age range of 25–73 years, either irradiated during head and neck cancer treatment ( n =3; all males aged 43, 68 and 73 years) or non-IR controls ( n =5; four males aged 29, 44, 58, 64 years and one female 25 years), were provided to Dr B. Baum by the Cooperative Human Tissue Network (CHTN), Mid-Atlantic Division, a National Cancer Institute supported resource. An exemption from the Office of Human Subjects Research at the National Institutes of Health was obtained as no patient identifiers were provided. This arrangement also met HIPAA (Health Insurance Portability and Accountability Act of 1996) privacy requirements. The CHTN requires us to state that other investigators may have received samples from these same tissue specimens. Thick cryosections (100 μM) of frozen tissue samples were used for staining to visualize the nerves in the tissue. The slices were immunostained as described above for whole-mount embryonic SMG staining. RNA was prepared from 3 × 50 μm 2 frozen sections from each biopsy sample. Two separate RNA pools were made from different levels in each biopsy, and qPCR reactions were performed from both pools from each sample with similar outcomes. The qPCR graphs in Fig. 4 are combined results from the three IR and three non-IR samples. Statistics Data were log transformed before all statistical analysis. We used GraphPad Prism 6 software (GraphPad Software Inc., CA). The Student’s t -test was used to compare two different groups, one-way analysis of variance with post hoc Dunnett’s test to compare more than two experimental groups and multiple unpaired t -tests were analysed by a false discovery rate approach where Q , the acceptable rate for false discoveries, was set to 5%. Graphs show the mean±s.d. How to cite this article: Knox S.M et al . Parasympathetic stimulation improves epithelial organ regeneration. Nat. Commun. 4:1494 doi: 10.1038/ncomms2493 (2013).